Mechanism of signal transduction of the LOV2-Jα photosensor fromAvena sativa Fusion proteins containing blue-light-activable protein domains possess great potential as molecular switches in cell signalling. This has recently been impressively demonstrated by connecting the light oxygen voltage LOV2-Jα-protein domain of A. sativa (AsLOV2-Jα) with the Rac1-GTPase, responsible for regulating the morphology and motility of metazoan cells. However, a target-oriented development of fusion proteins in conjunction with this photosensor is still very challenging, because a detailed understanding of its signal transduction pathway on a molecular level is still lacking. Here, we show through molecular dynamics simulation that, after formation of the cysteinyl-flavin mononucleotide (FMN) adduct, the signalling pathway begins with a rotational reorientation of the residue glutamine 1029 adjacent to the FMN chromophore, transmitting stress through the Iβ strand towards the LOV2-Jα interface. This then results in the breakage of two H-bonds, namely, glutamic acid 1034–Gln995 and aspartic acid (Asp) 1056–Gln1013, at opposite sides of the interface between the Jα helix and the LOV2 domain, ultimately leading to a disruption of Jα helix from the LOV2 core. Photoactivable fusion proteins possess great potential as photoenzymes or photoswitches in cell signalling [1] . By connecting a light-sensitive light oxygen voltage (LOV)-protein domain of phototropin1 from A. sativa (oat) to a Rac1 mutant, Wu et al . [2] , [3] have recently created a genetically encoded fusion protein that can reversibly be activated with blue light and be used to control cell movement. In the dark, this LOV domain interacts with a C-terminal α-helix (Jα) and, when fused to a target enzyme, sterically blocks effector protein binding. In biological systems, LOV domains are the light-sensitive part of plant phototropins. They absorb light through a flavin mononucleotide (FMN) cofactor, which leads to the formation of a covalent bond between the chromophore and a reactive cysteine residue of the apo protein. This triggers a signal in the attached serine/threonine kinase, leading to protein autophosphorylation [4] . Although tremendous progress has been accomplished on the elucidation of the primary photoreaction [5] , [6] and the characterization of the main intermediates of the photocycle [7] , [8] , [9] of LOV domains, the mechanism of signal transduction at the molecular level, involving signal propagation from the LOV2 domain to the Jα helix resulting in subsequent kinase activation, is still only poorly understood. In the past decade, several experimental works have attempted to clarify the response mechanism of phototropins to blue-light photoexcitation. To this end, major efforts were concentrated on the investigation of the dynamic changes of isolated LOV domains in the light state [4] , [10] . Studies of independent protein parts, however, can only provide limited information on the complex interaction mechanism taking place between the different structural elements of the full phototropin during the signal-transduction process. Harper et al . [11] first characterized the light-dependent changes of the AsLOV2-Jα photosensor ( Fig. 1a,b ) by solution NMR spectroscopy and found that the Jα helix plays a key role in kinase activation. From their results, they deduced that the photoinduced adduct formation in the LOV2 domain results in the disruption of the Jα helix from the Gβ-, Hβ- and Iβ strands, which in turn may trigger a signal in the kinase. To examine how the structural changes upon illumination are coupled to kinase activation, Harper et al . [12] in a subsequent work performed a series of point mutations along the Jα helix to disrupt its interaction with the LOV domain under dark-state conditions. Using NMR spectroscopy and limited proteolysis, they demonstrated that several of these mutations are able to displace the Jα helix from the LOV domain even in the absence of light. When placed into the full-length phototropin, these point mutations displayed constitutive kinase activation without illumination of the sample. These results indicate that unfolding of the Jα helix is the critical event in the regulation of the kinase signal. Recent crystallographic data from Halavaty and Moffat [13] on the AsLOV2-Jα photosensor also attributed the Jα helix with a predominant role in signal transduction. Although these studies clearly identified the C-terminal Jα helix to be responsible for communicating the signal to a downstream effector domain, it remained unclear how covalent adduct formation in the core triggers the α-helical unfolding on the surface of the domain. In a series of experimental and theoretical studies with LOV2 domains, a conserved glutamine residue, located on the Iβ strand in the immediate vicinity of the FMN-binding site, was found to change its H-bonding pattern with the FMN upon photoexcitation and was suspected to be involved in the transmission of the local stress to the surface of the LOV domain [4] , [10] , [14] , [15] . By designing point mutations of this glutamine residue and monitoring the effects on the LOV2 domain using ultraviolet–visible absorbance and circular dichroism spectroscopy, Nash et al . [16] recently confirmed that it plays a central role in both spectral tuning and signal propagation from the LOV2 core to the peripheral Jα helix. However, up to now, a detailed understanding of the spatio-temporal dynamics of the molecular processes involved in this critical event is still lacking. 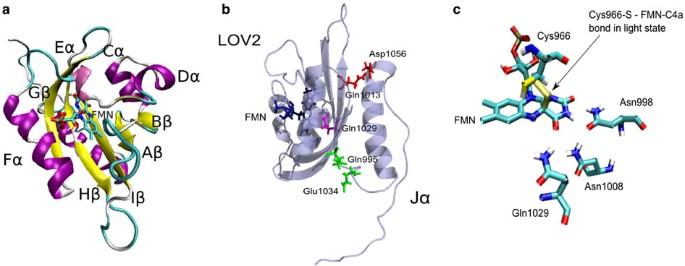Figure 1: Starting structures of the AsLOV2-Jα photosensor. (a) Dark-state solution structure of the AsLOV2-Jα system, refined through NMR measurements. (b) AsLOV2 protein core with the adjacent Jα helix and relevant amino acids (violet: Gln1029; red: Asp1056, Gln1013; green: Glu1034, Gln995). (c) Difference in the starting structures between dark- and adduct-state forms, structurally only differing with regard to the covalent bond of the CFN, and relevant amino acids surrounding the FMN chromophore (cyan: C-atom; red: O-atom; blue: N-atom; white: H-atom; brown: P-atom; yellow: S-atom). Figure 1: Starting structures of the AsLOV2-Jα photosensor. ( a ) Dark-state solution structure of the AsLOV2-Jα system, refined through NMR measurements. ( b ) AsLOV2 protein core with the adjacent Jα helix and relevant amino acids (violet: Gln1029; red: Asp1056, Gln1013; green: Glu1034, Gln995). ( c ) Difference in the starting structures between dark- and adduct-state forms, structurally only differing with regard to the covalent bond of the CFN, and relevant amino acids surrounding the FMN chromophore (cyan: C-atom; red: O-atom; blue: N-atom; white: H-atom; brown: P-atom; yellow: S-atom). Full size image In this study, we elucidate the early stages of the signal-transduction pathway of the AsLOV2-Jα photosensor at the molecular level, using the molecular dynamics (MD) simulation method. Our study shows that the initial process after formation of the Cys966-FMN adduct involves the breakage of an H-bond between the carbonyl oxygen FMN-C4=O and the amino group of Gln1029, followed by a rotational reorientation of its sidechain. This triggering event near the FMN chromophore initiates the creation of a new H-bond between Gln1029 and Asn1008, coupling the Iβ and Hβ strands together, and causes a progressive extension of the Iβ strand, transmitting stress towards the LOV2-Jα interface. The latter process then induces the breakage of H-bonds at opposite sides of the interface, involving an H-bond between Glu1034 on the Jα-Iβ linker and Gln995 on the Gβ strand, as well as another between Asp1056 at the C-terminal end of the Jα helix and Gln1013 on the Hβ strand. Ultimately, this leads to a disruption and partial unfolding of the Jα helix from the LOV core. Details of the simulation as well as of the generation of the starting structures of our dark- and adduct-state simulations ( Fig. 1c ) are given in the Methods. Wild-type AsLOV2-Jα photosensor We start the analysis of our simulation results by considering the spatio-dynamic behaviour of relevant amino acids near the FMN chromophore in the dark and adduct states. 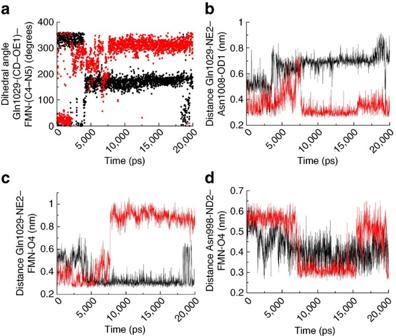Figure 2: Spatio-dynamic behaviour of amino acids near the FMN chromophore. Dihedral angle or distance of characteristic atoms on the FMN chromophore or on surrounding amino acids to atoms of neighbouring amino acid residues in the dark (black) and adduct (red) states (a) dihedral angle Gln1029-CD–Gln1029-OE1–FMN-C4–FMN-N5. (b) Distance Gln1029-NE2–Asn1008-OD1. (c) Distance Gln1029-NE2–FMN-O4. (d) Distance Asn998-ND2–FMN-O4. In Figure 2a, we draw the dihedral angle of the adduct state, enclosing the atoms Gln1029-CD, Gln1029-OE1, FMN-C4 and FMN-N5 as a function of simulation time. We observe that in the initial stage, the quantity fluctuates around an average value of 30°, followed after a simulation time of 2,500 ps by a sudden rotation of the angle of about 270° to a new average value of 300°. 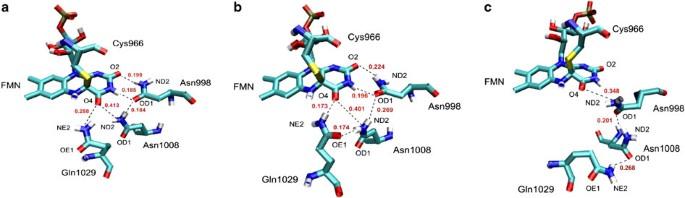Figure 3: Triggering event of the signalling pathway of the AsLOV2-Jα photosensor. Representative local configurations of amino acids Gln1029, Asn1008 and Asn998 surrounding the FMN chromophore at different simulation times, including H-bond distances in units of Å ((a) 0 ps, (b) 2,500 ps, (c) 8,000 ps). This rotational reorientation of the glutamine residue is visualized in Figure 3 , in which we compare the representative local configurations of the amino acids Gln1029, Asn1008 and Asn998 surrounding the FMN chromophore at different characteristic simulation times. In case of the configuration at 0 ps ( Fig. 3a ), the FMN-C4=O-carbonyl oxygen is twice H-bonded by the sidechains of Gln1029 and Asn1008, whereas the FMN-C2=O-carbonyl oxygen is twice H-bonded by the Asn998 and Gln970 sidechains. Comparing this configuration with the one at 2,500 ps ( Fig. 3b ), we see that the rotation of the dihedral angle of about 270° corresponds to a switch of the carbonyl oxygen of Gln1029-OE1 about the axis formed by the sidechain atoms Gln1029-NE2 and Gln1029-CD of the glutamine residue. This process initiates the release of amino acid Asn1008 through breakage of the H-bond between Gln1029 and Asn1008, as can be deduced from the increase in the distance between Gln1029-NE2 and Asn1008-OD1 in Figure 2b , triggered at the same simulation time. From this graph, we can further conclude that this distance undergoes a sudden drop to a value of about 3 Å at around 7,500 ps, which relates to the formation of a new H-bond between the amino group of Gln1029-NE2 and Asn1008-OD1 belonging to the Iβ and Hβ strands, respectively. The corresponding configuration is visualized in Figure 3c . We observe that the formation of a new H-bond causes a stable coupling between both β-strands, persisting over the remaining simulation time. We point out that this coupling process is consistent with the early stage of a β-sheet tightening process, observed in Fourier transform infrared spectroscopic experiments on LOV2 [17] , [18] and LOV2-Jα systems [19] . From the distances between Gln1029-NE2 and FMN-O4 in Figure 2c, as well as between Asn998-ND2 and FMN-O4 in Figure 2d , we see that the H-bond formation process goes along with an abrupt detachment of the residue Gln1029 from the FMN chromophore and a simultaneous stabilization of the local conformation through the creation of a new H-bond between Asn998-ND2 and FMN-O4, leaving the FMN-C4=O singly H-bonded with Asn998. This latter H-bond, however, is only transient and Asn998 can fluctuate back to its original position, as can be deduced from the subsequent jumps in Figure 2d at 17000 ps and 19,500 ps. In this context, it is worth mentioning that the glutamine residue adjacent to the FMN chromophore is highly conserved and has previously been suggested to be crucial for the signalling process of the LOV domains. Several early experimental studies on the isolated LOV2 domain suggested that the primary process after adduct formation involves the breakage of an H-bond between the glutamine residue and FMN-O4 [10] , possibly followed through rotation of its sidechain by the formation of a new H-bond with FMN-N5 [14] , [20] . In a later crystallographic study on the AsLOV2-Jα system, Halavaty and Moffat [13] proposed a local reorientation of the conserved glutamine, associated with a disruption of an H-bond between an asparagine and aspartic acid on the surface of the protein. In a series of spectroscopical investigations with point mutations of the LOV2-Jα system [16] , [21] , as well as the full-length phototropin [4] , it was demonstrated that this glutamine residue plays a central role in both spectral tuning and propagating the signal through the Iβ strand from the LOV core to the Jα helix, whereas its lack attenuates light-induced autophosphorylation of the phototropin. In a recent theoretical work on the isolated AsLOV2 domain, Freddolino et al . [15] deduced from MD simulations that adduct formation induces the breakage of an H-bond between the conserved glutamine and FMN-O4, followed by the creation of a new H-bond with FMN-N5. In addition, their simulation results suggested a second conformation, in which the glutamine interacted with neighbouring residues on the Iβ strand, leading to an increased mobility in the LOV2-Jα interface region. However, a clear molecular picture of the signalling process could not be established in this work, because of the neglect of the Jα helix. From our simulation results, we conclude that the primary steps after adduct formation involve the breakage of an H-bond between Gln1029-NE2 and FMN-O4, followed by a rotational reorientation of the glutamine residue Gln1029 and subsequent creation of a new H-bond between the amino group of Gln1029-NE2 and Asn1008-OD1. This latter process causes the coupling and tightening of the Iβ and Hβ strands. Moreover, it permits to propagate stress to the LOV2-Jα interface, which ultimately leads to the detachment of the Jα helix from the LOV2 domain, as we show in the following section. Figure 2: Spatio-dynamic behaviour of amino acids near the FMN chromophore. Dihedral angle or distance of characteristic atoms on the FMN chromophore or on surrounding amino acids to atoms of neighbouring amino acid residues in the dark (black) and adduct (red) states ( a ) dihedral angle Gln1029-CD–Gln1029-OE1–FMN-C4–FMN-N5. ( b ) Distance Gln1029-NE2–Asn1008-OD1. ( c ) Distance Gln1029-NE2–FMN-O4. ( d ) Distance Asn998-ND2–FMN-O4. Full size image Figure 3: Triggering event of the signalling pathway of the AsLOV2-Jα photosensor. Representative local configurations of amino acids Gln1029, Asn1008 and Asn998 surrounding the FMN chromophore at different simulation times, including H-bond distances in units of Å (( a ) 0 ps, ( b ) 2,500 ps, ( c ) 8,000 ps). 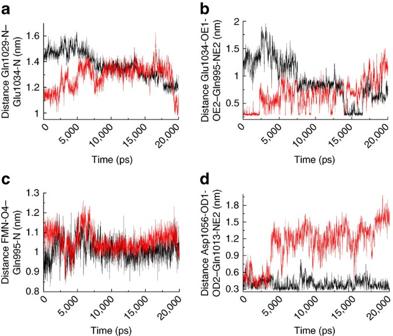Figure 4: Spatio-dynamic behaviour of amino acids at the LOV2-Jα interface. Interatomic distance from characteristic amino acids located on the interface between the Jα helix and the LOV2 core in the dark (black) and adduct (red) state (a) Gln1029-N–Glu1034-N. (b) Glu1034-OE1(OE2)–Gln995-NE2. (c) FMN-O4–Gln995-N. (d) Asp1056-OD1(OD2)–Gln1013-NE2. Full size image In Figure 4, we present data from our dark- and adduct-state simulations of characteristic interatomic distances of residues, located at the LOV2-Jα interface, as a function of time. The respective residues are depicted in Figure 1b . In Figure 4a, we first display the minimum distance between the backbone nitrogen atoms of the conserved glutamine residue Gln1029-N, which initially links the Iβ strand through its sidechain to the FMN-O4, and glutamate Glu1034-N, located on the Iβ strand in the linker region between the LOV2 core and the Jα helix. In the case of the adduct state, we observe starting from 2,500 ps a steady increase in the distance between both amino acids up to a maximum amount of 2 Å. This relates to the propagation of stress along the Iβ strand after the rotational reorientation of the Gln1029 sidechain, leading to a progressive extension of the backbone chain. From Figure 4b , we deduce that the latter process leads to the successive disruption of the H-bond between Glu1034-(OE1)OE2, located on the linker between the LOV2 core and the Jα helix, and the amino group of Gln995-NE2 on the Gβ strand. The release of the residue Glu1034 causes a perturbation of the Gβ backbone in the time range from 2,500 ps to 7,500 ps, as can be deduced from the oscillating distance between the backbone nitrogen atom Gln995-N and FMN-O4 in Figure 4c . However, afterwards, the distance re-adopts fluctuations around a similar average value as before the perturbation, which shows that overall the Gβ strand remains unaffected by this process. Next, we deduce from the strong jump of about 1 nm in the distance between Asp1056-OD1(OD2) and Gln1013-NE2, which can be observed at 3,000 ps in Figure 4d , that the cleavage of the H-bond between Glu1034 and Gln995 at 2,500 ps causes a subsequent breakage of the H-bond between Asp1056-OD1(OD2) and the amino group of Gln1013-NE2, located at the opposite end of the Jα helix and Hβ strand, respectively. By further considering the distance between Gln1029-NE2 and Asn1008-OD1 in Figure 2b , we clearly see that the rotational reorientation of Gln1029, which begins at 2,500 ps, results in the subsequent disruption of the H-bond between Asp1056 and Gln1013. In this situation, the Jα helix starts successively to disrupt from one end of the LOV2 domain. At 17,000 ps, we observe an accelerated increase in the distance between Asp1056-OD1(OD2) and Gln1013-NE2. This coincides with the full disruption of the H-bond between Glu1034 and Gln995, characterized through the rise in the distance between Glu1034-(OE1)OE2 and Gln995-NE2 in Figure 4b at the same simulation time. The latter process ultimately leads to the complete detachment of the Jα helix from the LOV2 domain, which is followed by a relaxation of the β-strands. This conclusion can easily be drawn from the drops in the distance at 18,000 ps between the backbone nitrogen atoms Gln1029-N and Glu1034-N on the Iβ strand in Figure 4a , as well as the distance between the backbone nitrogen Gln995-N on the Gβ strand and FMN-O4 in Figure 4c . Figure 4: Spatio-dynamic behaviour of amino acids at the LOV2-Jα interface. Interatomic distance from characteristic amino acids located on the interface between the Jα helix and the LOV2 core in the dark (black) and adduct (red) state ( a ) Gln1029-N–Glu1034-N. ( b ) Glu1034-OE1(OE2)–Gln995-NE2. ( c ) FMN-O4–Gln995-N. ( d ) Asp1056-OD1(OD2)–Gln1013-NE2. Full size image In their seminal paper on phototropin switches, Harper et al . [11] compared the dark- and adduct-state 3D-HNCO spectra of the AsLOV2-Jα system, using the minimum chemical-shift-difference method to quantify the spectral changes. Within the LOV2 core, they observed large differences for the residues close to the FMN chromophore, as well as for the ones on the Gβ, Hβ and Iβ strands. Significant perturbations were also observed at sites on the Eα helix and the Jα helix over 15 Å away from the FMN chromophore. They concluded from their work that the structural changes induced by the formation of the cysteinyl-FMN (CFN) adduct propagate through the LOV domain, ultimately causing the disruption of the Jα helix. To determine which of the protein segments at the LOV2-Jα interface could be critical in the detachment process, they further created a truncated protein lacking the last 24 residues of the AsLOV2-Jα system (AsLOV2ΔJα), starting from residue Glu1053 up to the end of the Jα helix. This deletion removes a key portion of the C-terminal Jα helix, including the H-bond-forming residue Asp1056. The comparison of the dark-state 15 N/ 1 H-HSQC-spectra of the AsLOV2-Jα- and AsLOV2ΔJα systems revealed significant chemical-shift differences for residues located inside the core of the protein domains. Further removal of C-terminal residues, starting from Asp1038, leaving only the LOV2 core (AsLOV2Δ), produced no additional spectral changes in the dark-state spectra. These results indicate that the Jα helix possesses a critical interaction with the LOV2 core in the protein part containing Asp1056 that is removed by truncation. 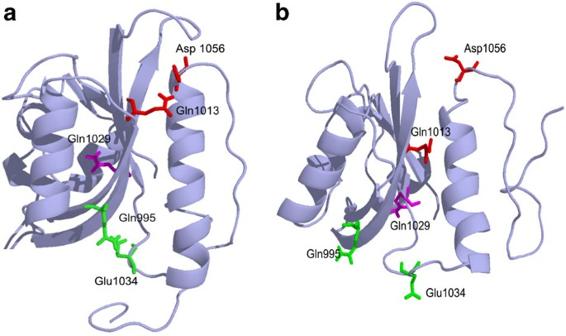Figure 5: Final secondary structures of the dark and adduct states of the AsLOV2-Jα photosensor. Secondary structures at a simulation time of 20 ns from the dark (a) and adduct (b) states of the AsLOV2-Jα system with relevant amino acids (violet: Gln1029; red: Asp1056, Gln1013; green: Glu1034, Gln995). In Figure 5, we present secondary structures of the AsLOV2-Jα system in the dark (a) and adduct (b) states at the final simulation time of 20 ns. In the figure, we highlight the H-bond between Gln995 and Glu1034 (green), as well as the one between Asp1056 and Gln1013 (red), in addition to residue Gln1029 (violet). By comparing both structures, we clearly see that the structural changes at the Hβ and Iβ strands upon adduct formation go along with the breakage of H-bonds at the LOV2-Jα interface. Moreover, we recognize that the Jα helix in case of the adduct state is partially unfolded at its C-terminal end. We note that in this segmental part of the Jα helix, starting from lysine (Lys) 1049, the sequence is more conserved among phototropins than at the N-terminal end of the Jα helix and the Iβ-Jα loop [13] , which indicates that this part of the protein might be important in the signal-transduction pathway. 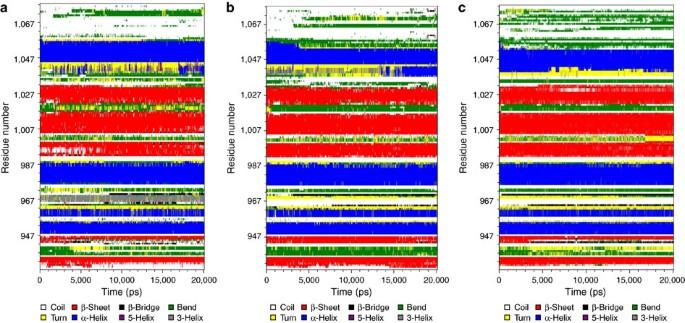Figure 6: Secondary structure analysis of the wild-type AsLOV2-Jα photosensor and its Gln1029Asn mutant. Secondary structure analysis from simulations of the wild-type AsLOV2-Jα system in the dark (a) and adduct (b) states, as well as of its Gln1029Asn mutant in the adduct state (c). This observation is further confirmed in Figure 6 , in which we present the secondary structure analysis of our simulations of the AsLOV2-Jα system in the dark (a) and adduct (b) states. Whereas in the dark-state simulation the Jα helix remains stable over the entire production run, we see that the Jα helix in the adduct state simulation partially looses its helical structure at a simulation time of 3,000 ps, starting from Asn1054 up to the end of the Jα helix. This unfolding process clearly correlates with the breakage of the H-bond at the same simulation time between Asp1056 on the Jα helix and Gln1013 on the Hβ strand, as shown in Figure 4d . In addition, in the secondary structure analysis, we observe at around 17,000 ps an increase in the length of the Jα helix through the formation of an additional helical element between residues Asp1038 and Glu1043. This event coincides with the full disruption of the H-bond between Glu1034 and Gln995 at the same simulation time, as can be deduced from Figure 4b . Finally, we observe in case of the adduct state a stabilization of the smaller β-strands at the outer peripheral of the LOV2 domain, denoted as Aβ and Bβ strands, which may contribute to an increase in the hydrophobicity of the LOV2 domain at the interface and accelerate the detachment of the Jα helix from the LOV2 domain. The rest of the secondary structure remains essentially unaffected through the adduct formation. It is worth emphasizing in this context that our conclusions concord well with the NMR measurements of Harper et al . [11] on the AsLOV2-Jα system in the dark and adduct states. In their study, it was demonstrated that the photosensor undergoes a selective unfolding of the C-terminal Jα helix upon adduct formation, implicating that the conformational changes in the LOV domain must be sufficiently destabilizing in order to displace the Jα helix without globally unfolding the LOV core. These findings were confirmed in a series of consecutive experimental works on the same system, using various spectroscopic techniques [16] , [19] . To investigate the role of the unfolding process of the Jα helix after its detachment from the LOV2 core, Harper et al . [12] created point mutations that disrupted the Jα helix in the absence of light. From these experiments, they concluded that the unfolding of the Jα helix is the critical event for triggering the kinase activity. Figure 5: Final secondary structures of the dark and adduct states of the AsLOV2-Jα photosensor. Secondary structures at a simulation time of 20 ns from the dark ( a ) and adduct ( b ) states of the AsLOV2-Jα system with relevant amino acids (violet: Gln1029; red: Asp1056, Gln1013; green: Glu1034, Gln995). Full size image Figure 6: Secondary structure analysis of the wild-type AsLOV2-Jα photosensor and its Gln1029Asn mutant. Secondary structure analysis from simulations of the wild-type AsLOV2-Jα system in the dark ( a ) and adduct ( b ) states, as well as of its Gln1029Asn mutant in the adduct state ( c ). Full size image Gln1029Asn mutant of the AsLOV2-Jα photosensor To demonstrate how the precise knowledge of the mechanism of signal transduction can be used to influence the transduction pathway and engineer the signal activity of the AsLOV2-Jα system, we designed a point mutant, replacing Gln1029 with its methylene-less counterpart asparagine, and investigated the effect of this substitution on the mechanism of signal transduction. 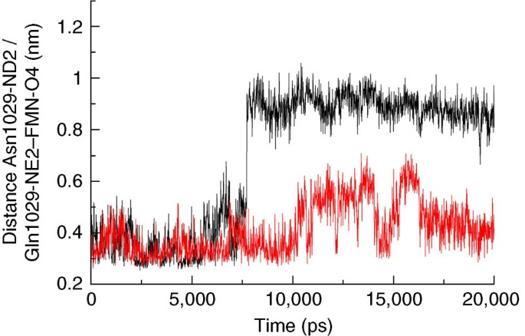Figure 7: Spatio-dynamic behaviour of the conserved glutamine of the AsLOV2-Jα photosensor versus the corresponding asparagine of its Gln1029Asn mutant. Distance between Gln1029-NE2 and FMN-O4 in the wild-type AsLOV2-Jα system (black) compared to the distance between Asn1029-ND2 and FMN-O4 in the AsLOV2-Jα-Gln1029Asn mutant (red). Both photosensors are in their adduct-state form. In Figure 7, we compare the distance between Gln1029-NE2 and FMN-O4 in the wild-type AsLOV2-Jα system with the corresponding distance in the mutant between Asn1029-ND2 and FMN-O4. We observe that the mutant does not show any major jump in the distance, which might indicate an abrupt detachment of Asn1029-ND2 on the Iβ strand from the FMN chromophore, as observed in case of the wild type for the distance between Gln1029-NE2 and FMN-O4 at 7,500 ps. To assess the effect of the mutation on the light-induced structural changes and thus the signal intensity, we next compared the secondary structure analysis of the wild-type AsLOV2-Jα system and its Gln1029Asn mutant in the adduct state in Figure 6b,c . We see that in case of the asparagine mutant, the light-induced structural changes, observed in the residue range of the Jα-helix, are reduced compared to the wild-type AsLOV2-Jα system. This indicates that the signal activity is damped because of the substitution and that Gln1029 plays a central role in the signal propagation from the LOV2 core to the Jα helix in the wild-type system, sensitively affecting the intensity of the signal. We note that these results agree well with recent experimental measurements of Nash et al . [16] on the same system, using a combination of ultraviolet–visible absorbance-, circular dichroism- and NMR spectroscopy. These authors found that mutation at this site causes a significant reduction of the light-induced structural changes of the protein domain, while maintaining its photocycling capabilities. Moreover, they concluded, to explain the slightly accelerated dark-state recovery kinetics of the mutant with respect to the wild-type AsLOV2-Jα system, that the mutant retains the H-bond between the amide group of Asn1029 and FMN-O4, observed in the dark-state, also in the adduct-state form. Thus, we see that a precise knowledge of the mechanism of signal transduction allows to engineer the signal activity of the AsLOV2-Jα system by altering the degree of light-induced structural changes through the introduction of mutations, and demonstrates the predictive power of our simulation procedure. Figure 7: Spatio-dynamic behaviour of the conserved glutamine of the AsLOV2-Jα photosensor versus the corresponding asparagine of its Gln1029Asn mutant. Distance between Gln1029-NE2 and FMN-O4 in the wild-type AsLOV2-Jα system (black) compared to the distance between Asn1029-ND2 and FMN-O4 in the AsLOV2-Jα-Gln1029Asn mutant (red). Both photosensors are in their adduct-state form. Full size image Our study demonstrates that the signal-transduction pathway after adduct formation of the AsLOV2-Jα photosensor begins with altering the H-bond network by means of a rotational reorientation of a conserved glutamine residue adjacent to the FMN chromophore, inducing the coupling of the Iβ and Hβ strands, as well as the propagation of stress through the Iβ strand to the LOV2-Jα interface. The stress then causes the breakage of an H-bond at the interface between residues on the C-terminal end of the Jα helix and the Hβ strand, as well as another H-bond between residues on the Jα-Iβ linker and the Gβ strand. Ultimately, this leads to a disruption of the Jα helix from the LOV2 core and a partial unfolding of the Jα helix. We anticipate that the elucidation of the AsLOV2-Jα signal-transduction pathway at a molecular level presented in this work will provide new perspectives for the creation of novel fusion proteins in combination with the AsLOV2-Jα photosensor. As demonstrated on the example of its asparagine mutant AsLOV2-Jα-Gln1029Asn, this knowledge can be used to engineer novel fusion proteins with optimized light-induced response, which might open new avenues for allosteric control of protein activity in living cells [22] , [23] , [24] , [25] . Generation of starting structures As a starting structure for our dark-state simulation, we used the dark-state solution structure of the LOV2-Jα protein domain from phototropin1 of A. sativa AsLOV2-Jα of Harper et al ., [11] which is a modelled structure refined with nuclear Overhauser effect (NOE) values originating from NMR measurements. To create the initial structures of our adduct-state simulations for both the wild-type AsLOV2-Jα system and its Gln1029Asn mutant, we used the dark-state solution structure previously mentioned and generated a cysteinyl-FMN (CFN) adduct by forming a covalent bond between Cys966-S and FMN-C4a. Our assumption is that the process of adduct formation is fast, compared with the overall relaxation of the system, and that the structure does not change during this short time span. In Figure 1a we visualize the secondary structure of the LOV2-Jα domain and FMN in its binding pocket, whereas in Figure 1b we display the Jα helix aggregated to the LOV2 core. The latter figure contains the amino acids relevant for signal transduction, discussed in the further development. In Figure 1c, we visualize the difference in the starting structures between the dark- and adduct-state forms, which structurally only differ with regard to the covalent bond of the CFN. Simulation details To resolve the signal-transduction pathway from the AsLOV2-Jα photosensor at a molecular level, we generated MD trajectories making use of the GROMACS MD simulation package version 3.3, in conjunction with the GROMOS43A1 forcefield [26] , to describe the interactions, unless explicitly specified otherwise. This widely used forcefield has been tested against NMR spectroscopic data in case of the hen egg white globular protein lysozyme in water by Soares et al . [27] and has been found to reproduce its solution structure and conformational behaviour very well. In a recent work, Todorova et al . [28] performed extensive MD simulations on the 51-amino-acid protein, insulin, and subjected the GROMOS43A1 forcefield to a systematic comparison against other popular biomolecular forcefields, including the CHARMM27-, AMBER03-, OPLS- and GROMOS53A6 forcefields. They analysed in detail the effect of each forcefield on the conformational evolution and structural properties of the protein and compared the results with the available experimental data. They observed that each forcefield favours different structural trends. Moreover, they found that the united-atom forcefield GROMOS43A1, together with the CHARMM27 forcefield, delivered the best description of the experimentally observed dynamic behaviour of the chain B of insulin. In our simulations, we used, in addition, full particle-mesh-Ewald (PME) electrostatics with a Coulomb cutoff of 1.4 nm and computed the van der Waals (vdW) interactions, using a shift function with a cutoff of 1.4 nm. We placed the protein into a cubic box with a boxlength of 7.4 nm and filled it with SPC water and seven sodium ions to neutralize the system. To generate an isothermal–isobaric ensemble with a temperature of 300 K and a pressure of 1 atm, the system was equilibrated for 1 ns. During this phase, every part of the system was coupled to a Nosé-Hoover thermostat and a Parrinello-Rahman barostat [29] . We then performed a production run of 20 ns, in which the protein and FMN were decoupled from the thermostat, whereas the solvent and ions remained coupled. We call this technique the non-invasive thermostating technique, which allows the protein to sample configurations far from equilibrium and to follow its natural dynamics under solvent-mediated thermostating control. For the numerical integration of the equations of motion, we used the leapfrog integrator with a timestep of 1 fs. To describe the interactions of the CFN, we used the parameters of Neiss and Saalfrank [30] , which were determined from B3LYP-6-31G * calculation results and through comparison with similar groups in the forcefield to reach consistency. The reliability of the parametrization of both CFN and FMN was tested and confirmed by these authors on the LOV2 domain from Adiantum capillus-veneris without the Jα helix [30] . How to cite this article: Peter, E. et al . Mechanism of signal transduction of the LOV2-Jα photosensor from Avena sativa . Nat. Commun. 1:122 doi: 10.1038/ncomms1121 (2010).